Structure of ERK2 bound to PEA-15 reveals a mechanism for rapid release of activated MAPK ERK1/2 kinases are the principal effectors of a central signalling cascade that converts extracellular stimuli into cell proliferation and migration responses and, when deregulated, can promote cell oncogenic transformation. The scaffolding protein PEA-15 is a death effector domain protein that directly interacts with ERK1/2 and affects ERK1/2 subcellular localization and phosphorylation. Here, to understand this ERK1/2 signalling complex, we have solved the crystal structures of PEA-15 bound to three different ERK2 phospho-conformers. The structures reveal that PEA-15 uses a bipartite binding mode, occupying two key docking sites of ERK2. Remarkably, PEA-15 can efficiently bind the ERK2 activation loop in the critical Thr-X-Tyr region in different phosphorylation states. PEA-15 binding triggers an extended allosteric conduit in dually phosphorylated ERK2, disrupting key features of active ERK2. At the same time PEA-15 binding protects ERK2 from dephosphorylation, thus setting the stage for immediate ERK activity upon its release from the PEA-15 inhibitory complex. The RAS–RAF–MEK–ERK signalling axis represents a core regulatory cascade governing the fundamental cellular processes of cell proliferation, migration and invasion [1] , [2] , [3] . Components of this pathway, particularly the RAS small GTPase and the RAF serine/threonine kinase, are among the most frequently mutated genes in human cancer and also represent key targets for cancer therapy [4] . Binding of GTP-loaded RAS family GTPases [5] activates RAF, which phosphorylates and activates the dual specificity mitogen-activated protein (MAP) kinase kinase, MEK1. In turn, MEK1 activates ERK (extracellular signal-regulated kinase)1/2 through dual phosphorylation of a critical Thr-X-Tyr motif in the ERK activation loop. This cascade is further controlled by scaffolding proteins such as Kinase Suppressor of Ras (KSR), which recruits multiple components of the pathway to facilitate efficient signal transduction culminating in ERK1/2 activation [2] , [6] . Activated ERK1/2 phosphorylate cytosolic substrates but also translocate to the nucleus, where they phosphorylate an array of critical targets to promote proliferation and differentiation [7] , [8] . While the RAS–RAF–MEK cascade represents the main ERK1/2 upstream regulatory cascade, control of ERK1/2 function can also occur at the level of the kinase itself [2] . PEA-15 (15 kDa phosphoprotein enriched in astrocytes) is a widely expressed protein that efficiently regulates ERK1/2 despite consisting of only a death effector domain (DED) and a short carboxy-terminal tail. By directly binding ERK1/2, PEA-15 is capable of inhibiting ERK1/2 activity and preventing their translocation to the nucleus, therefore, regulating the two most pivotal aspects of ERK signalling [9] , [10] , [11] , [12] . The designation of PEA-15 as an ERK inhibitor is based on multiple studies showing that PEA-15 inhibits the classical outcomes of ERK signalling. For example, in neuroblastomas, PEA-15 impairs cell migration [13] , and in astrocytic tumours inversely correlates with tumour malignancy [14] . Binding of PEA-15 to ERK has also been reported to impair tumour cell invasion and to contribute to Ras induced cell senescence [15] , [16] . Additionally, PEA-15 can directly inhibit ERK-mediated phosphorylation of the classical ERK1/2 substrates ELK-1 and ETS-1 in in vitro assays [17] . However, recent studies reporting oncogenic functions of PEA-15 hint at a regulatory role rather than a solely inhibitory impact on ERK1/2 signalling. These oncogenic functions of PEA-15 include potentiating H-Ras-mediated epithelial cell transformation and protecting glioblastoma cells from glucose deprivation-induced cell death [18] , [19] . Thus, PEA-15 appears to efficiently suppress ERK1/2 function, but in certain settings can also function to promote tumour growth. Here we present three structures of PEA-15 bound to different phosphorylated states of ERK2, which provide the first structural insight into an ERK2 regulator complex. Our study reveals how PEA-15 has evolved to act as an ERK1/2 repressor that, in its inhibitory complex with the kinase, induces an accumulation of phosphorylated ERK and thus sets the stage for ERK pathway activation. PEA-15 targets the two main ERK-docking sites, using a ‘minimal’ D-peptide-docking site interaction and a ‘regulatory’ DEF-docking site interaction. The structures also show that as part of the regulatory DEF-docking site interaction, PEA-15 directly binds the ERK activation loop, which is accompanied by an extended network of allosteric changes. Altogether, the molecular mechanism of the ERK–PEA-15 interaction transforms the view of PEA-15 from a mere ERK1/2 inhibitor to a sophisticated ERK1/2 regulator and reveals a plethora of ERK2 regulatory elements. Structure of the PEA-15–ERK2 complex To obtain insight into the mechanism underlying ERK1/2 regulation by PEA-15, we sought to obtain the crystal structure of the PEA-15-ERK complex by using several combinations of full-length PEA-15 with different activation states and phosphomimetic mutants of ERK2 in crystallization trials. After testing these in a broad array of crystallization screens, we succeeded in crystallizing an activation loop phosphomimetic (T185E) mutant of ERK2 (residues 8–360) in complex with full-length PEA-15 and solved the structure of the complex at a resolution of 3.2 Å ( Fig. 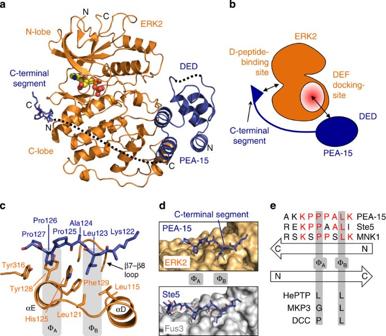Figure 1: PEA-15 interacts with ERK2 using a bipartite binding mode. (a) Structure of the PEA-15–ERK2 complex. Shown is the structure of ERK2 (orange) with bound ADP (yellow) and the DED and C-terminal segment of PEA-15 in blue (regions not defined by electron density are schematically indicated by dotted lines; N and C termini of the DED and C-terminal segment are indicated). (b) Cartoon illustration of the PEA-15–ERK2 complex. PEA-15 utilizes a bipartite binding mode to occupy the two main regulatory sites of ERK2. The DED of PEA-15 (blue) occupies the ERK2 DEF-docking region (red), while the C-terminal segment of PEA-15 occupies the D-peptide-binding site. (c) Detailed view of the PEA-15 C-terminal segment (residues 122–127; blue sticks) binding to the D-peptide-binding site on ERK2 (orange). Interface sidechains and secondary structural elements are labelled. (d) The PEA-15 C-terminal segment binds ERK2 (top) in a manner similar to the binding of the scaffold protein Ste5 to the yeast MAP kinase Fus3 (bottom; residues 306–314, PDB: 2f49). (e) Conservation between PEA-15, Ste5 and MNK1. Schematic illustration of binding modes (see alsoSupplementary Figs S2 and S3). Displayed are the respective D-peptide sequences with residues occupying the ΦAand ΦBsites annotated. Relative directionality and key interaction residues are depicted in comparison with the canonical D-peptide binding mode. 1a , Table 1 ). In the structure, the crystallographic asymmetric unit shows a subarrangement of two ERK2 molecules bound to two molecules of PEA-15 ( Supplementary Fig. S1a ). In the most completely defined subarrangement, electron density was observed for PEA-15 residues 1–30 and 37–86 (defining the DED), and residues 122–127 (defining the PEA-15 C-terminal interaction segment). Residues 31–36 of the DED and the linker region (87–121) connecting the C-terminal interaction segment with the PEA-15 DED lacked electron density and were not included in the model. ERK2 electron density was observed for residues 9–357, with an adenosine diphosphate (ADP) nucleotide occupying the nucleotide-binding site of the kinase. To identify the biologically relevant assembly, we examined the complex in solution using analytical ultracentrifugation and size-exclusion chromatography ( Supplementary Fig. S1b,c ). This revealed an assembly consistent with one ERK2 molecule bound to one PEA-15 molecule in solution. Thus, we inferred that an arrangement consisting of an ERK2 molecule in complex with the PEA-15 DED and C-terminal segment as depicted in Fig. 1a constitutes the PEA-15–ERK2 complex. Figure 1: PEA-15 interacts with ERK2 using a bipartite binding mode. ( a ) Structure of the PEA-15–ERK2 complex. Shown is the structure of ERK2 (orange) with bound ADP (yellow) and the DED and C-terminal segment of PEA-15 in blue (regions not defined by electron density are schematically indicated by dotted lines; N and C termini of the DED and C-terminal segment are indicated). ( b ) Cartoon illustration of the PEA-15–ERK2 complex. PEA-15 utilizes a bipartite binding mode to occupy the two main regulatory sites of ERK2. The DED of PEA-15 (blue) occupies the ERK2 DEF-docking region (red), while the C-terminal segment of PEA-15 occupies the D-peptide-binding site. ( c ) Detailed view of the PEA-15 C-terminal segment (residues 122–127; blue sticks) binding to the D-peptide-binding site on ERK2 (orange). Interface sidechains and secondary structural elements are labelled. ( d ) The PEA-15 C-terminal segment binds ERK2 (top) in a manner similar to the binding of the scaffold protein Ste5 to the yeast MAP kinase Fus3 (bottom; residues 306–314, PDB: 2f49). ( e ) Conservation between PEA-15, Ste5 and MNK1. Schematic illustration of binding modes (see also Supplementary Figs S2 and S3 ). Displayed are the respective D-peptide sequences with residues occupying the Φ A and Φ B sites annotated. Relative directionality and key interaction residues are depicted in comparison with the canonical D-peptide binding mode. Full size image Table 1 Data collection and refinement statistics. Full size table PEA-15 occupies key ERK2-docking sites in a bipartite manner The complex structure reveals that PEA-15 employs a bipartite binding mode involving both its DED and the segment within its C-terminus to interact with ERK2 ( Fig. 1b ), which is in line with earlier biochemical analysis of the ERK2–PEA-15 interaction [11] , [17] . Generally, bipartite binding enhances the affinity of individually weaker interactions and allows for greater binding specificity. Beyond the advantages inherent to bipartite binding, PEA-15 applies this mode of binding to occupy two key docking sites on ERK2, namely the D-peptide-binding site and the DEF interaction site ( Fig. 1b ) (ref. 20 ). The ERK2 D-peptide-binding site is targeted by proteins that contain a distinctive D-motif (also termed DEJL/docking site for E RK and J NK, L XL or KIM/kinase interaction motif) [20] . These proteins include substrates, but also upstream kinases, scaffolding proteins and phosphatases [21] . The D-peptide-binding site is the only binding site on ERK2 that has been structurally characterized at high resolution before this study, with five structures now available of peptide fragments from ERK2 partners bound to the ERK2 D-peptide-binding site [22] , [23] , [24] , [25] . The other site on ERK1/2 that is targeted by PEA-15 is known as the DEF-docking site (docking site for ERK, FxF), due to its characteristic ability to bind proteins that contain a consensus motif with two phenylalanine residues separated by one amino acid (FxF) [26] . This docking site is key to ERK1/2’s interaction with substrates and scaffold proteins, as well as components of the nuclear transport machinery that are crucial for ERK1/2 nuclear translocation. Thus, utilizing a bipartite binding mode that engages both sites ( Fig. 1b ) enables PEA-15 to inhibit ERK1/2 function and explains its general capacity to inhibit ERK enzymatic activity ( Supplementary Fig. S2a ) [17] , as well as its tumour suppressor role [13] , [14] , [15] , [16] . PEA-15 uses a minimal inverted D-peptide binding mode Closer examination of the interaction between the C-terminal segment of PEA-15 (residues 122–127) and the D-peptide-binding site of ERK2 ( Fig. 1c , Supplementary Fig. S2b,c ) shows that this segment of PEA-15 adopts an extended conformation, occupying the groove between helices αD and αE and the β7-β8 turn on the C-terminal lobe of ERK2. Comparison with the crystal structures of peptides from deleted in colorectal cancer (DCC), MAP kinase phosphatase and hematopoietic tyrosine phosphatase bound to ERK2 shows that PEA-15 occupies this site in a non-canonical manner ( Supplementary Fig. S3 ). Intriguingly, PEA-15 utilizes a minimal D-peptide interaction consensus motif (see also below) that binds in the opposite direction to that observed in the above structures [17] , [21] . In detail, the Φ A pocket on the ERK2 D-peptide-binding site is occupied by Pro126 of PEA-15, with Pro127 extending the hydrophobic interaction by packing against Tyr128 and Tyr316 at the edge of the pocket. The Φ B pocket created by ERK2 residues Leu115, Leu121 and Phe129 is filled by Leu123 of PEA-15 ( Fig. 1c ). Analysis over a wider array of MAP kinase–D-peptide complexes shows that the PEA-15 C-terminal segment is almost identical to the binding-motif used by the yeast scaffold protein Ste5 to regulate its target kinase Fus3 ( Fig. 1d ) [27] . Very recently, the structures of MNK1 and RSK1 D-peptides have been solved in complex with ERK2 and also exhibit a reverse D-peptide binding mode [25] ( Fig. 1e ; Supplementary Fig. S2d ). Intriguingly, the MNK1 D-peptide shows remarkable similarity in the backbone conformation of residues 435–439 when compared with the PEA-15 C-terminal segment. However, the MNK1 peptide interaction also includes an extended helical-binding element (MNK1 residues 439–450), ( Supplementary Fig. S2d ), which buries an additional 380 Å 2 of interaction surface, resulting in a tight interaction with a dissociation constant of 700 nM (ref. 25 ). In contrast, the much smaller PEA-15 ERK D-peptide-binding interaction is rather weak, with a dissociation constant of 18 μM ( Supplementary Fig. S2e ). Thus, PEA-15 utilizes a minimal inverse D-peptide that blocks the hydrophobic portion of the D-peptide-binding site with moderate affinity, consistent with regulatory rather than constitutive inhibition of ERK2. In line with this, mutation of L123K in the C-terminal segment of PEA-15 substantially weakens the binding to ERK2 ( Fig. 2d ), and results in the failure of the PEA-15 L123K mutant to prevent ERK nuclear translocation ( Fig. 2e ). Taken together, the minimal reverse D-peptide binding of PEA-15 demonstrates the structural adaptability of the D-peptide-docking site and raises the possibility that other ERK1/2-binding partners employ this mode of binding, which may be a hallmark of moderate affinity regulatory interactions with this site. 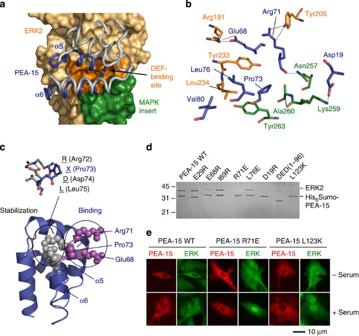Figure 2: The PEA-15 DED interacts with the ERK2 DEF-docking site. (a) PEA-15 DED (worm representation) binding to ERK2 (surface). The PEA-15 DED is rendered in grey with interacting helices α5-α6 coloured blue, while binding residues of ERK2 residing in the DEF-binding region and the MAP kinase insert are coloured orange and green, respectively. (b) Detailed view of the PEA-15–DEF-binding-site interaction (PEA-15 residues are depicted in blue, ERK2 DEF-binding site and MAP kinase insert residues are rendered orange and green, respectively). (c) The DED RXDL motif is not involved in binding. The PEA-15 DED (blue ribbon) is depicted with Arg72, Asp74 and Leu75 of the RXDL motif displayed as grey spheres (detailed view shown in stick representation above). The RXDL residues do not participate in the interaction with ERK2 but function to stabilize the neighbouring residues Glu68, Arg71 and Pro73 (magenta), which do interact with ERK2. (d) Mutational analysis of PEA-15 residues involved in ERK2 binding. Recombinantly expressed and purified His6-tagged PEA-15 proteins were incubated with untagged ERK2 and captured on Ni-NTA resin, which after wash steps was subjected to SDS–PAGE. Protein bands were visualized with Coomassie blue. (e) Effect of PEA-15 WT and mutants deficient in ERK2 binding on nuclear translocation of ERK2. NIH3T3 cells expressing WT and mutant EGFP-PEA-15 (pseudocoloured in red) were immunolabelled for ERK1/2 (pseudocoloured in green). A representative scale bar of 10 μm is displayed below. PEA-15 is always located in the cytosol. In serum-starved cells, ERK2 is retained in the cytosol in the presence of PEA-15 WT and to a lesser extent in the presence of the mutant PEA-15. In serum-stimulated cells, strong nuclear translocation of ERK2 can be observed in the presence of the R71E and L123K PEA-15 mutants compared with PEA-15 WT. Figure 2: The PEA-15 DED interacts with the ERK2 DEF-docking site. ( a ) PEA-15 DED (worm representation) binding to ERK2 (surface). The PEA-15 DED is rendered in grey with interacting helices α5-α6 coloured blue, while binding residues of ERK2 residing in the DEF-binding region and the MAP kinase insert are coloured orange and green, respectively. ( b ) Detailed view of the PEA-15–DEF-binding-site interaction (PEA-15 residues are depicted in blue, ERK2 DEF-binding site and MAP kinase insert residues are rendered orange and green, respectively). ( c ) The DED RXDL motif is not involved in binding. The PEA-15 DED (blue ribbon) is depicted with Arg72, Asp74 and Leu75 of the RXDL motif displayed as grey spheres (detailed view shown in stick representation above). The RXDL residues do not participate in the interaction with ERK2 but function to stabilize the neighbouring residues Glu68, Arg71 and Pro73 (magenta), which do interact with ERK2. ( d ) Mutational analysis of PEA-15 residues involved in ERK2 binding. Recombinantly expressed and purified His 6 -tagged PEA-15 proteins were incubated with untagged ERK2 and captured on Ni-NTA resin, which after wash steps was subjected to SDS–PAGE. Protein bands were visualized with Coomassie blue. ( e ) Effect of PEA-15 WT and mutants deficient in ERK2 binding on nuclear translocation of ERK2. NIH3T3 cells expressing WT and mutant EGFP-PEA-15 (pseudocoloured in red) were immunolabelled for ERK1/2 (pseudocoloured in green). A representative scale bar of 10 μm is displayed below. PEA-15 is always located in the cytosol. In serum-starved cells, ERK2 is retained in the cytosol in the presence of PEA-15 WT and to a lesser extent in the presence of the mutant PEA-15. In serum-stimulated cells, strong nuclear translocation of ERK2 can be observed in the presence of the R71E and L123K PEA-15 mutants compared with PEA-15 WT. Full size image The DED of PEA-15 occupies the ERK2 DEF-docking site PEA-15 utilizes its DED to bind the ERK2 DEF-docking site [26] , [28] , and our structure provides the first high-resolution structural insight into an ERK2–DEF site interaction ( Fig. 2a ). It is also the first structural view of the interaction of a death domain protein with a kinase. The PEA-15–ERK2 structure shows that the DED of PEA-15 utilizes helices α5 and α6 and the linker between the two helices to bind ERK2 residues residing in helices αG and αEF ( Fig. 2a ). This interaction network is supported by ERK2 residues from the first helix of the MAP kinase insert, which is characteristic of MAP kinases ( Fig. 2a ). In detail, the DEF-docking site interaction surface utilized by PEA-15 is generated by ERK2 Tyr233 and Leu234 and the DEF-docking site region proper, as well as the stem of Lys259, Ala260 and Tyr263 from the MAP kinase insert, which together form a hydrophobic surface to accommodate Pro73, Leu76 and Val80 of PEA-15. This patch is completed by polar interactions between residues Asp19, Glu68 and particularly Arg71 (see also Fig. 3 ) from PEA-15 and Arg191, Tyr205, Asn257 and Lys259 from ERK2 ( Fig. 2b ). The DEF docking interaction is crucial for PEA-15 function, including its ability to sequester ERK1/2 and prevent its translocation to the nucleus [29] , [30] , [31] . Accordingly, the mutation of PEA-15 Arg71 at the centre of the interface abrogates cytoplasmic retention of ERK2 by PEA-15 ( Fig. 2d ) [10] , [11] . 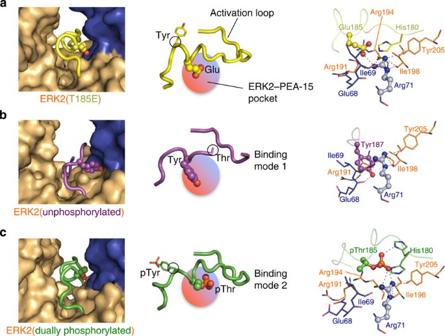Figure 3: PEA-15 binds the ERK2 activation loop in two distinct modes. (a) PEA-15 binding to ERK2(T185E). Left: Close-up of the PEA-15–ERK2 composite surface pocket (orange/blue) accepting Glu185 and the activation loop in a helical conformation (yellow). Middle: Schematic of the activation loop showing Tyr187 and Glu185 and the activation loop conformation in relation to the composite pocket. Right: Detailed view of interactions surrounding Glu185 (ERK2 residues coloured orange and PEA-15 residues blue, and activation loop residues rendered in yellow). (b,c) Analogous representations of the PEA-15–ERK2 pocket accommodating (b) unphosphorylated ERK2 activation loop and (c) the dually phosphorylated activation loop (activation loop residues are coloured purple and green, respectively). Figure 3: PEA-15 binds the ERK2 activation loop in two distinct modes. ( a ) PEA-15 binding to ERK2(T185E). Left: Close-up of the PEA-15–ERK2 composite surface pocket (orange/blue) accepting Glu185 and the activation loop in a helical conformation (yellow). Middle: Schematic of the activation loop showing Tyr187 and Glu185 and the activation loop conformation in relation to the composite pocket. Right: Detailed view of interactions surrounding Glu185 (ERK2 residues coloured orange and PEA-15 residues blue, and activation loop residues rendered in yellow). ( b , c ) Analogous representations of the PEA-15–ERK2 pocket accommodating ( b ) unphosphorylated ERK2 activation loop and ( c ) the dually phosphorylated activation loop (activation loop residues are coloured purple and green, respectively). Full size image PEA-15 DED RXDL motif serves to position binding residues The PEA-15–ERK2 structure also shows that the DEF-docking site interaction does not directly involve residues Arg72, Asp74 or Leu75, which constitute the so called RXDL motif of the PEA-15 DED. Generally, the RXDL motif is a hallmark of DED proteins and is conserved among members of this family. The function of this motif has remained unclear, although it has been proposed to have a role in the interaction with binding partners [32] . Surprisingly, PEA-15 residues Glu68, Arg71 and Leu76, which are key for the interaction with ERK2, are not part of the RXDL motif but reside directly beside the residues constituting the motif ( Fig. 2c ). Instead, Arg72, Pro73, Asp74, Leu75 (RXDL) partake in interactions within the DED of PEA-15, thus reinforcing the local structure of the domain. Hence, the role of the RXDL motif lies not in binding but in stabilization of the α5-loop-α6 region, thus properly positioning the critical binding residues of PEA-15 ( Fig. 2c ). The PEA-15 DED directly binds the ERK2 activation loop An unexpected aspect of PEA-15 interaction with the ERK2–DEF site is that the ERK2 activation loop directly participates in the binding interface. This is surprising, given that kinase activation loops are commonly characterized by a large degree of plasticity [33] , [34] , [35] , which could potentially make them a destabilizing factor in binding interactions. However, the structure reveals that in the PEA-15–ERK2 complex the region around the Glu185 of the activation loop is ‘captured’ by a binding pocket created by residues from both PEA-15 and ERK2 ( Fig. 3a ). As outlined above, Glu185 was used as phosphomimetic for pThr185 of the ERK2 Thr-X-Tyr motif. The PEA-15–ERK2 composite pocket captures the Glu185 phosphomimetic utilizing an arginine stretch that includes ERK2 residues Arg191, Arg194 and particularly Arg71 from PEA-15, which is the most central residue of this interaction ( Fig. 3a ). As a consequence of this capture, the activation loop adopts a helical conformation and is fully defined in the PEA-15–ERK2 complex ( Fig. 3a ). This mechanism explains how PEA-15 is able to engage a threonine-phosphorylated ERK2 activation loop. Yet, PEA-15 exhibits similar binding affinities for all phosphorylation states of ERK2 ( Supplementary Fig. S4 ), raising the question of how PEA-15 interacts with the unphosphorylated and dually phosphosphorylated ERK2 kinase. PEA-15 captures the activation loop in two distinct modes To answer this question we solved the structures of the PEA-15 DED (residues 1–96) bound to unphosphorylated and dually phosphorylated ERK2 at resolutions of 1.8 and 1.9 Å, respectively ( Supplementary Figs S5a,b and S6 ). These structures show a similar overall interaction by the PEA-15 DED ( Supplementary Fig. S5c,d ), but importantly reveal how PEA-15 is able to avidly bind ERK2 regardless of its phosphorylation status by using two distinct binding modes to capture the activation loop. The structure of PEA-15 in complex with the unphosphorylated ERK2 shows that the composite pocket formed by PEA-15 and the DEF-docking site of ERK2 is able to also bind the unphosphorylated activation loop, but by interacting with Tyr187 from the Thr-X-Tyr motif ( Fig. 3b ). The binding of Tyr187 is accompanied by a register shift of two amino acids within the activation loop, compared with the binding of the phosphomimetic Glu185. As a consequence, the activation loop following Thr185 adopts an extended rather than helical conformation in this binding mode (mode 1) and the N-terminal portion of the activation loop (residues 179–184) is partially disordered. Furthermore, Arg71 of PEA-15 now undergoes a stacking interaction with the aromatic side chain of Tyr187 to anchor the activation loop ( Fig. 3b , right panel). The structure of dually phosphorylated ERK2 in complex with PEA-15 demonstrates mode 2 of activation loop binding, which is highly similar to that observed in the structure of PEA-15 in complex with the phosphomimetic Glu185 mutant. The activation loop adopts the same helical conformation, with the phosphate moiety of pThr185 binding to the composite pocket formed by ERK2 and PEA-15 ( Fig. 3c ). PEA-15 binding reveals extended allosteric conduit in ERK2 Comparison of dually phosphorylated ERK2 in its unbound- and PEA-15-bound forms [33] also reveals that the binding of the PEA-15 DED triggers a network of allosteric changes in ERK2. Firstly, PEA-15 counteracts the interaction of the two phosphate groups of pThr185 and pTyr187 with their binding pockets in ERK2 ( Fig. 4a ), which leads to the rearrangement of the activation loop described above. This modification in turn leads to an extended network of short- and long-range allosteric rearrangements in the kinase ( Fig. 4a , Supplementary Movie ). In detail, Glu68 of PEA-15 displaces Tyr233 towards the αEF helix and dislodges pTyr187 from its pocket on ERK2. In parallel, Arg71 of PEA-15 directly sequesters pThr185, as well as Tyr205, which flips away from its previous location lining the pThr185 pocket in ERK2 ( Fig. 4a , Supplementary Fig. S7 ). 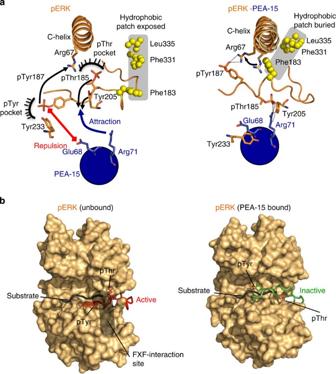Figure 4: PEA-15-ERK2 regulatory interaction. (a) PEA-15 binding triggers concerted allosteric changes in phospho-ERK2. Left: Unbound ERK2 before PEA-15 binding. Phospho-Thr185 and phospho-Tyr187 are anchored into defined pockets in phosphorylated ERK2 (PDBid:2erk). Upon binding, PEA-15 Glu68 repels phospho-Tyr187 and Tyr233, while Arg71 of PEA-15 attracts phospho-Thr185 and Tyr205 (indicated by red and blue arrows). Right: Conformations observed in the PEA-15–phosphor-ERK2 complex. In the complex, PEA-15 Arg71 forms a direct salt bridge with pThr185 and coordinates Tyr205, while pTyr187 interacts with Arg67 located in the αC-helix. As a consequence, the activation loop adopts a helical conformation that is accompanied by long-range allosteric changes (see alsoSupplementary Movie 1) in catalytic elements such as the αC-helix, as well as the burial of a distal hydrophobic patch (residues displayed in yellow spheres). (b) PEA-15 ‘regulatory’ DEF interaction differs from- and precludes substrate-like binding. Comparison of the activation loop conformations of unbound dually phosphorylated ERK2 (left panel, red; PDB: 2erk) and PEA-15-bound phospho-ERK2 (right panel, green). The position of a putative peptide substrate (black; depicting residues P−3 to P+3 of a substrate from a cAMP-dependent protein kinase substrate complex/PDB:1L3R) is also depicted. Additionally the putative FxF-binding region on ERK2 is indicated for unbound phospho-ERK2 (grey area; see alsoSupplementary Fig. S8). This region has been shown to capture a characteristic FxF sequence motif downstream of the phosphorylation site in key ERK substrates. Figure 4: PEA-15-ERK2 regulatory interaction. ( a ) PEA-15 binding triggers concerted allosteric changes in phospho-ERK2. Left: Unbound ERK2 before PEA-15 binding. Phospho-Thr185 and phospho-Tyr187 are anchored into defined pockets in phosphorylated ERK2 (PDBid:2erk). Upon binding, PEA-15 Glu68 repels phospho-Tyr187 and Tyr233, while Arg71 of PEA-15 attracts phospho-Thr185 and Tyr205 (indicated by red and blue arrows). Right: Conformations observed in the PEA-15–phosphor-ERK2 complex. In the complex, PEA-15 Arg71 forms a direct salt bridge with pThr185 and coordinates Tyr205, while pTyr187 interacts with Arg67 located in the αC-helix. As a consequence, the activation loop adopts a helical conformation that is accompanied by long-range allosteric changes (see also Supplementary Movie 1 ) in catalytic elements such as the αC-helix, as well as the burial of a distal hydrophobic patch (residues displayed in yellow spheres). ( b ) PEA-15 ‘regulatory’ DEF interaction differs from- and precludes substrate-like binding. Comparison of the activation loop conformations of unbound dually phosphorylated ERK2 (left panel, red; PDB: 2erk) and PEA-15-bound phospho-ERK2 (right panel, green). The position of a putative peptide substrate (black; depicting residues P−3 to P+3 of a substrate from a cAMP-dependent protein kinase substrate complex/PDB:1L3R) is also depicted. Additionally the putative FxF-binding region on ERK2 is indicated for unbound phospho-ERK2 (grey area; see also Supplementary Fig. S8 ). This region has been shown to capture a characteristic FxF sequence motif downstream of the phosphorylation site in key ERK substrates. Full size image The activation loop rearrangement is accompanied by several conformational adjustments of key functional elements of the kinase, such as the Glycine-rich loop and C-helix (see Supplementary Movie 1 ). In parallel, a large exposed hydrophobic patch distal from the catalytic center of the kinase (formed by residues Phe183, Phe331 and Leu335) becomes buried upon PEA-15 binding ( Fig. 4 ). These rearrangements reveal an interconnected conformational conduit that is linked to the PEA-15–ERK2 DEF-binding site interaction and may also be utilized by other binding partners for ERK regulation. The conduit spans from the nucleotide-binding region of ERK2 through the central groove to the outlined hydrophobic patch, which has been speculated to mediate ERK2 dimerization events and other protein interactions [36] , [37] , [38] . PEA-15 binding defines a regulatory ERK DEF site interaction The allosteric conduit triggered by PEA-15 in combination with the activation loop engagement revealed by our ERK2–PEA-15 complex structures suggests a new view of ERK DEF-binding site interactions that distinguishes between ‘substrate like’ and ‘regulatory’ type interactions. Firstly, PEA-15 binding causes the activation loop in ERK2 to adopt an inactive conformation despite being dually phosphorylated. This becomes evident when a putative substrate, derived from the structure of substrate-bound cyclic adenosine monophosphate-dependent protein kinase [39] , is overlaid onto dually phosphorylated ERK2 unbound or bound to PEA-15 (ref. 33 ) ( Fig. 4b ). The overlay shows that in PEA-15-bound ERK2 the pThr and pTyr, together with the helical conformation of the activation loop, completely occlude the substrate-binding region normally available in phospho-ERK2. Secondly, as outlined above, the term DEF-docking site was initially based on its ability to interact with substrates containing a FxF motif downstream of the substrate Ser/Thr residue. While no structure of an FxF-type substrate-bound to ERK is available, various groups have predicted features of this interaction [26] , [28] , [40] . The surface pockets highlighted in Fig. 4b and Supplementary Fig. S8 are based on a model by Turk and colleagues [28] and illustrate the two key binding regions in ERK2 that are predicted to accommodate the Phe moieties of FxF substrate motifs. However, PEA-15 does not contain a FxF motif and the binding of the PEA-15 DED occurs only in the general area of these pockets. In fact, only Leu234 and Tyr263 from the predicted FxF-binding pockets make a direct hydrophobic contact with PEA-15 ( Fig. 2b ), while Tyr 231 and pTyr 185 reorient as part of the allosteric PEA-15 interaction mechanism ( Supplementary Fig. S8 ). Thus, PEA-15 binding partially dismantles the binding pocket for the first Phe of the motif, in addition to relocating the activation loop. These features suggest the existence of two types of DEF interactions. One represents a classic FxF-type DEF interaction, in which substrates bind to the defined FxF pockets of dually phosphorylated ERK1/2 in a catalytically competent conformation. The second type of DEF-site interaction mediates the regulatory binding of ERK effectors. In this case, the binding partners utilize an interaction pattern that differs from the FxF substrate-type binding. Instead, these factors use the DEF-docking site to alter the ERK1/2 activation loop, which may also facilitate its phosphorylation or dephosphorylation. PEA-15 protects phospho-ERK1/2 from dephosphorylation We next sought to investigate the physiological consequences of the ability of PEA-15 to capture the Thr-X-Tyr activation loop of ERK in its different phosphorylation states. First, we examined the effect of PEA-15 binding on ERK2 activation by its upstream kinase MEK1 ( Fig. 5a , Supplementary Fig. S9a–c ). Our in vitro kinase assays show that PEA-15 reduces the rate of MEK1-dependent ERK2 phosphorylation, but it nevertheless allows accumulation of fully phosphorylated ERK2. In fact we find that at a concentration of 17 μM, which may reflect MEK–KSR–ERK activation platforms, MEK1 is able to displace PEA-15 ( Supplementary Fig. S9d ). Taken together, these results are consistent with earlier in vitro studies that define PEA-15 as an inhibitor of ERK1/2 phosphorylation [10] , but suggest that PEA-15 is a permissive regulator rather than inhibitor of ERK2 phosphorylation. 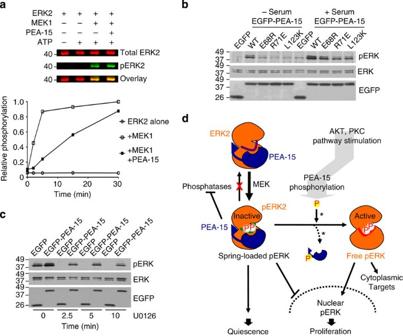Figure 5: PEA-15 leads to the stabilization of spring-loaded ERK1/2. (a) PEA-15-bound ERK2 is permissive to phosphorylation by MEK1. Anin vitrophosphorylation assay of ERK2 shows a decreased rate of ERK phosphorylation but still allows for accumulation of phospho-ERK2. Time course of ERK2 phosphorylation by constitutive active MEK1 (quantified, bottom) and 30 min end points of the assay (LICOR visualization, top). (b) Wild-type PEA-15, but not binding interface mutants, leads to enrichment of dually phosphorylated ERK1/2 in both unstimulated and serum-stimulated cells. Extracts from cells expressing wild-type PEA-15, or ERK1/2-binding interface mutants of PEA-15, were probed for dually phosphorylated ERK2. (c) PEA-15 protects phospho ERK from dephosphorylation. HEK293 cells expressing EGFP-PEA-15 or control vector were stimulated with serum and subsequently treated with 10 μM U0126 to inhibit MEK1 for the indicated times. Extracts were analysed at the indicated time points by western blotting with the indicated antibodies. (d) Accumulation of halted, ‘spring-loaded’ phospho-ERK1/2 highlights the dual nature of PEA-15. Schematic illustrating the cellular consequences of the PEA-15-ERK regulatory mechanism, which allows for integration of diverse pathways and signalling outcomes (asterisks next to the arrows describing the release of phosphorylated PEA-15 from ERK1/2 indicate that the mechanism of this release is not known and may involve displacement through an additional unknown protein)17. Figure 5: PEA-15 leads to the stabilization of spring-loaded ERK1/2. ( a ) PEA-15-bound ERK2 is permissive to phosphorylation by MEK1. An in vitro phosphorylation assay of ERK2 shows a decreased rate of ERK phosphorylation but still allows for accumulation of phospho-ERK2. Time course of ERK2 phosphorylation by constitutive active MEK1 (quantified, bottom) and 30 min end points of the assay (LICOR visualization, top). ( b ) Wild-type PEA-15, but not binding interface mutants, leads to enrichment of dually phosphorylated ERK1/2 in both unstimulated and serum-stimulated cells. Extracts from cells expressing wild-type PEA-15, or ERK1/2-binding interface mutants of PEA-15, were probed for dually phosphorylated ERK2. ( c ) PEA-15 protects phospho ERK from dephosphorylation. HEK293 cells expressing EGFP-PEA-15 or control vector were stimulated with serum and subsequently treated with 10 μM U0126 to inhibit MEK1 for the indicated times. Extracts were analysed at the indicated time points by western blotting with the indicated antibodies. ( d ) Accumulation of halted, ‘spring-loaded’ phospho-ERK1/2 highlights the dual nature of PEA-15. Schematic illustrating the cellular consequences of the PEA-15-ERK regulatory mechanism, which allows for integration of diverse pathways and signalling outcomes (asterisks next to the arrows describing the release of phosphorylated PEA-15 from ERK1/2 indicate that the mechanism of this release is not known and may involve displacement through an additional unknown protein) [17] . Full size image Additionally, we found that PEA-15 overexpression leads to an accumulation of phosphorylated ERK1/2 in transiently transfected cells ( Fig. 5b ), in agreement with previous studies [18] , [41] . We also observed this accumulation in the absence of growth factor stimulation while PEA-15 interface mutants fail to propagate this effect ( Fig. 5b ). This observation suggests that PEA-15 protects phospho-ERK1/2 from dephosphorylation. To investigate this function of PEA-15, we examined its effect on the progressive decline of phospho-ERK1/2 following block of MEK activity. We measured phospho-ERK1/2 levels in the presence or absence of overexpressed PEA-15 in cells treated with the MEK inhibitor U0126 for various periods of time ( Fig. 5c ). The results show that, indeed, PEA-15 provides prolonged protection of phospho-ERK1/2 from dephosphorylation in serum-stimulated HEK293 cells treated with U0126 as compared with control cells where ERK1/2 phosphorylation is rapidly lost. The physiological outcome of the multifaceted binding mechanism applied by PEA-15 is an accumulation of a ‘spring-loaded’ phospho-ERK2 in complex with PEA-15. This accumulation occurs not only when upstream components of the ERK pathway are activated, but also under unstimulated conditions. However, even though ERK bound to PEA-15 is phosphorylated, its activation loop is held in an inactive conformation ( Fig. 4b ) and its nuclear transport is blocked. Consequently, in this scenario PEA-15 inhibits the activity of ERK1/2, proliferative signals are suppressed, and PEA-15 acts as tumour suppressor ( Fig. 5d ). However, the regulatory character of the PEA-15 ERK interaction allows PEA-15 to be released from ERK2. This release is reported to involve phosphorylation of PEA-15 Ser104/Ser116 (refs 42 , 43 ), yet occurs by an unknown mechanism because phosphorylation of PEA-15 has no direct effect on ERK binding [17] . Regardless of the mechanism of PEA-15 release, its consequence is that ‘spring-loaded’ phospho-ERK1/2 can now promptly adopt its default active conformation without further need for phosphorylation by upstream kinases ( Fig. 5d ). The released phospho-ERK1/2 will then phosphorylate their cytosolic substrates and translocate to the nucleus to phosphorylate nuclear substrates, inducing transcription and ultimately proliferation. Among the kinases that have been reported to phosphorylate PEA-15 on Ser104/Ser116 are protein kinase C, CaMKII and AKT (refs 42 , 43 ). Thus PEA-15 can link different pathways to ERK1/2 and, as in the case of AKT or protein kinase C, enhance their oncogenic effect. Importantly, the mechanism applied by PEA-15 also explains how ERK1/2 phosphorylation can be uncoupled from its signalling outcome [44] . While ERK1/2 phosphorylation is frequently used as marker for malignancy, the mechanism utilized by PEA-15 suggests that clinical testing strategies considering PEA-15 levels and phosphorylation, as well as a readout of ERK1/2 activity, can provide a more powerful prognostic tool than simply ERK1/2 phosphorylation levels [42] . In summary, the structural information from the PEA-15-ERK complex demonstrates that PEA-15 acts as an efficient mechanism-based regulator that employs known, as well as novel MAP kinase regulatory features. PEA-15 uses a bipartite binding mode and captures different activation states of ERK2 to suppress and direct the ultimate outcome of the ERK-signalling pathway. The structural features of this regulation provide remarkable insight into the inner workings of ERK1/2 kinase function, which involve a previously unidentified allosteric network. They also provide mechanistic insight into how a tumour suppressor can lead to an enrichment of phospho-ERK1/2, potentially priming the cell for a rapid activation of ERK1/2 by signalling pathways that target PEA-15. Protein expression and purification For crystallization Human ERK2 (Uniprot: P28482) residues 8–360 was cloned into a modified pET-LIC vector (kindly gifted by the Netherlands Cancer Insitute (NKI) Protein Facility with funding from grant no. 175.010.2007.012) incorporating an N-terminal His 6 tag and 3C protease cleavage site. To prepare dually phosphorylated ERK2 this construct was coexpressed with constitutively active MEK1 from pETDuet-ACYC in Escherichia coli , while unphosphorylated kinase was prepared by coexpression of YopH tyrosine phosphatase to minimize ERK2 autophosphorylation [45] . Full-length human PEA-15 (Uniprot: Q15121 residues 1–130) for crystallization was expressed from pET28b. All biophysical and biochemical experiments were performed using full-length ERK2 and PEA-15 expressed from a modified pET vector incorporating an N-terminal His 6 -tag and SUMO1 fusion protein. Treatment of these proteins with SENP1 protease yielded species with no residually amino acids for ERK2 (1–360) and a single additional glycine residue for PEA-15 in order to facilitate protease cleavage. The DED construct of PEA-15 for crystallization (residues 1–96) was also produced as a SUMO-fusion protein. All mutagenesis was performed using QuikChange site-directed mutagenesis. All proteins were initially purified by Ni 2+ affinity chromatography, and purified to homogeneity after cleavage with respective proteases using anion-exchange (Source Q 10/10) and size-exclusion (Superdex-200) chromatographies. Isolated proteins and complexes were flash frozen for storage in 10 mM HEPES (7.6), 100 mM NaCl and 0.5 mM tris-(2-carboxyethyl)phosphine. Crystallization For crystallization ERK2 T185E (8–360) and full-length PEA-15 were combined at high concentration and the complex was purified by size-exclusion chromatography at a protein concentration of ~20 mg ml −1 . Initial crystals of ERK2 T185E bound to full-length PEA-15 were grown by sitting drop vapour diffusion using a precipitant condition containing 0.1 M Bis-Tris (pH 5.5) and 2.0 M ammonium sulphate. These crystals diffracted anisotropically to 4 Å in the best dimension, and were improved by cycles of additive screening and soaking with nucleotides. Final crystals were grown from a condition containing 0.1 M Bis-Tris (pH 5.5), 1.8 M ammonium sulphate and 3% sucrose, soaked with 2 mM ADP for ~15 min in mother liquor, and cryoprotected by transferring to mother liquor containing 20% glycerol before freezing in a nitrogen cryostream. Purified unphosphorylated, and dually phosphorylated, ERK2 (8–360) were each mixed with PEA-15 (1–96) at equimolar ratios, concentrated to ~15 mg ml −1 and directly subjected to crystallization screening. Diffraction quality crystals of unphosphorylated ERK2–PEA-15 DED grew from a condition containing 0.2 M sodium malonate and 20% PEG 3350 (measured pH 5.5). Crystals of the dually phosphorylated ERK2 complex grew from 0.2 M potassium phosphate monobasic and 20% w/v Polyethylene glycol 3,350 (measured pH 5.0). Both crystal types were transferred to mother liquor containing 15% glycerol for cryoprotection before freezing. Structure determination Final diffraction data for all crystals was collected at National Synchrotron Light Source beamline X29 and processed using XDS [46] and SCALA [47] . The structure of the ERK2 T185E–PEA-15 complex was solved by molecular replacement in Phaser [48] using the structure of dually phosphorylated ERK2 (PDBid: 2erk) with the activation loop deleted as a search model. PEA-15 was successfully located using an edited poly-alanine model of the DED from MC159 (PDBid: 2bbr) as a search model. The overall structure was iteratively built and refined using Refmac5 (ref. 49 ) and COOT [50] . Structures of the complex between un- or dually phosphorylated ERK2 with the PEA-15 DED were solved by independent searches for the individually chains from the above structure, with the activation loop of ERK2 deleted from search models. In each crystal the asymmetric unit contained one molecule of PEA-15 bound to ERK2, and a second ERK2 polypeptide not bound to PEA-15. Isothermal titration calorimetry and analytical ultracentrifugation Isothermal titration calorimetry (ITC) was carried out using a MicroCal iTC200 calorimeter. PEA-15 full-length or fragments thereof (200–500 μM) were injected into ERK2 variants (20–50 μM) in a matched buffer containing 10 mM HEPES (7.6), 100 mM NaCl and 0.5 mM Tris-(2-carboxyethyl)phosphine. AMP-PNP (2 mM) was incorporated into the buffer of the diluent kinase to mimic the physiological presence of nucleotide. Analytical ultracentrifugation sedimentation equilibrium experiments were performed in a ProteomeLab XL-I (BeckmanCoulter) analytical ultracentrifuge with protein in the same buffer used for ITC. Analysis was done using HeteroAnalysis software (by J.L. Cole and J.W. Lary, University of Connecticut; http://www.biotech.uconn.edu/auf/ ). ERK2 activation assays Activation of ERK2 by MEK1 in vitro was performed using purified MEK1-R4F [51] purified with a C-terminal His 6 -tag. Combinations of ERK2 (5 μM), MEK1 (0.5 μM) and PEA-15 (10 μM) were incubated in a buffer containing 25 mM HEPES (pH 7.5), 100 mM NaCl, 20 mM MgCl 2 , 2 mM dithiothreitol, and 0.5 mM EGTA, with adenosine triphosphate (5 mM) added to initiate reactions. At indicated time points samples were removed, combined with SDS–polyacrylamide gel electrophoresis (PAGE) sample buffer and boiled to terminate the reaction. Following electrophoreses and western blotting, transferred proteins were probed with mouse derived α-ERK2 and rabbit α-phospho-ERK2 antibodies (both from Cell Signaling Technology). Detection was performed using LICOR IRDye α-mouse and α-rabbit secondary antibodies. PEA-15 inhibition assay of ERK2 activity ADP-glo assays (Promega) were performed to measure kinase activity of activated ERK2 in the presence and absence of PEA-15. Reactions were carried out in an identical buffer to the ERK2 activation assays described above. ERK2 (0.4 μM) was incubated with MBP (50 μM) and adenosine triphosphate (50 μM) with/without PEA-15 (5 μM) at room temperature for 30 min. Amounts of generated ADP were measured through luminescence according to the manufacturers' instructions in 384-well plates. In vitro binding assays between PEA-15 and ERK2 Untagged full-length ERK2 was isolated as described above in the protein expression and purification section; namely expressed as a His-Sumo-fusion protein, cleaved from the His-Sumo tag and finally purified using anion-exchange chromatography. Wild-type His-Sumo-PEA-15, or mutants thereof, were expressed as described above and purified via Ni- affinity chromatography. After eluation His-Sumo-PEA-15 proteins were incubated with an excess (~2:1) of the untagged ERK2 wt protein for 25 min at room temperature and then applied to Ni-NTA beads. After wash steps using a 10 mM Tris (pH 8.0), 100 mM NaCl, 10% glycerol, 10% sucrose and 2 mM dithiothreitol containing 30 mM imidazole, the Ni-NTA beads were mixed with SDS–PAGE sample buffer and subjected to SDS–PAGE. Protein bands were visualized using Coomassie staining. Characterization of ERK2–PEA-15 regulation in cells For immunoblotting, HEK 293 cells were cultured in DMEM supplemented with 10% fetal bovine serum (FBS) and penicillin/streptomycin and transiently transfected with EGFP or EGFP-tagged PEA-15 plasmids using Lipofectamine 2000 (Invitrogen). Twenty-four hours after transfection, the cells were starved in DMEM with 0.2% FBS for 18 h. The cells were then stimulated for 45 min with 20% FBS or maintained in 0.2% FBS and then lysed in modified RIPA buffer (150 mM NaCl, 50 mM Tris, pH 7.5 with 1% Triton X-100, 0.5% Na deoxycholate, 0.1% SDS, 2 mM EDTA, 1 mM sodium orthovanadate, 1 mM sodium fluoride, aprotinin, leupeptin, pepstatin 1 μg ml −1 each and 1 mM phenylmethylsulphonyl fluoride) and centrifuged at 16,000 g for 15 min at 4 °C. Total extracts were resolved by SDS–PAGE and transferred to PVDF membranes (Millipore) and then probed by immunoblotting with anti-phospho-ERK1/2 (Thr202/Tyr204) and anti-ERK1/2 antibodies (Cell Signaling; 1:50 dilution). Expression of transfected EGFP-PEA-15 was assessed by immunoblotting with an anti-GFP antibody (GeneTex; 1:2,500 dilution). After primary antibody incubation, membranes were incubated with an horseradish-conjugated anti-rabbit antibody (Millipore; 1:5,000 dilution) and a chemiluminescence system (GE Healthcare Life Sciences) was used for detection. To assess ERK dephosphorylation in the presence of PEA-15, HEK 293 cells transfected with either EGFP or PEA-15 WT were starved overnight. The cells were then stimulated with 20% FBS for 30 min to increase pERK levels, treated with 10 μM of the MEK inhibitor U0126 for different time periods, and lysed in modified RIPA buffer. For immunocytochemistry, NIH3T3 cells were cultured in DMEM (Cellgro, Mediatech) supplemented with 10% FBS and penicillin/streptomycin, and were transiently transfected with EGFP or EGFP-PEA-15 plasmids using Lipofectamine 2000 (Invitrogen). Fifteen hours after transfection, the cells were trypsinyzed and plated on glass coverslips coated with fibronectin (10 μg ml −1 ; Millipore). Twenty-four hours after transfection, the cells were starved in DMEM with 0.2% FBS for 18 h. The cells were then stimulated for 3 h with 20% FBS or maintained in 0.2% FBS and then fixed with 4% formaldehyde and permeabilized in 0.5% Triton X-100 in PBS. After a 30 min incubation with 10% normal goat serum in PBS at room temperature, the cells were incubated overnight at 4 °C with anti-ERK1/2 antibody (Cell Signaling; 1:50 dilution) in 10% normal goat serum in PBS. After PBS washes, the cells were incubated for 1 h at room temperature with the secondary anti-rabbit antibody conjugated with Alexa Fluor 568 (Invitrogen; 1:200 dilution). Nuclei were counterstained with 4′,6-diamidino-2-phenylindole (Sigma; 1:5,000) and the cells were mounted in ProLong Gold antifade reagent (Invitrogen). Accession codes: Atomic coordinates and structure factors have been deposited in the Protein Data Bank under accession codes 4IZ5 ((ERK2 T185E)–PEA-15), 4IZ7 (Non-phosphorylated ERK2–PEA-15(1–96)) and 4IZA (Dually phosphorylated ERK2–PEA-15(1–96)). How to cite this article: Mace, P.D. et al . Structure of ERK2 bound to PEA-15 reveals a mechanism for rapid release of activated MAPK. Nat. Commun. 4:1681 doi: 10.1038/ncomms2687 (2013).